The TFEB orthologue HLH-30 regulates autophagy and modulates longevity inCaenorhabditis elegans Autophagy is a cellular recycling process that has an important anti-aging role, but the underlying molecular mechanism is not well understood. The mammalian transcription factor EB (TFEB) was recently shown to regulate multiple genes in the autophagy process. Here we show that the predicted TFEB orthologue HLH-30 regulates autophagy in Caenorhabditis elegans and, in addition, has a key role in lifespan determination. We demonstrate that hlh-30 is essential for the extended lifespan of Caenorhabditis elegans in six mechanistically distinct longevity models, and overexpression of HLH-30 extends lifespan. Nuclear localization of HLH-30 is increased in all six Caenorhabditis elegans models and, notably, nuclear TFEB levels are augmented in the livers of mice subjected to dietary restriction, a known longevity-extending regimen. Collectively, our results demonstrate a conserved role for HLH-30 and TFEB in autophagy, and possibly longevity, and identify HLH-30 as a uniquely important transcription factor for lifespan modulation in Caenorhabditis elegans . Aging is modulated by multiple conserved signal transduction pathways, such as the insulin/insulin-like growth factor-1 (IGF-1) and target of rapamycin (TOR) signalling pathways. Studies in model organisms, including the nematode Caenorhabditis elegans , have identified key regulatory roles for several transcription factors in these pathways [1] . However, the degree to which these distinct longevity pathways converge on common downstream mechanisms remains an important topic of investigation. Macroautophagy (hereafter referred to as autophagy) is a cellular recycling process that has emerged as a crucial mechanism for lifespan extension in many different species [2] . During autophagy, cytosolic components are sequestered in vesicles called autophagosomes, which then fuse with lysosomes, allowing the contents to be enzymatically degraded and recycled. Notably, long-lived C. elegans mutants with reduced insulin/IGF-1 signalling, TOR signalling, germline signalling, food intake or mitochondrial respiration, all exhibit increased levels of autophagy and require autophagy genes for lifespan extension [3] . However, the mechanism(s) by which these long-lived animals regulate the autophagy process is not fully understood. We recently reported that the forkhead transcription factor PHA-4/FOXA regulates the expression of several genes important for autophagy in response to germline removal or TOR inhibition in C. elegans [4] . Moreover, PHA-4/FOXA and autophagy genes are essential for lifespan extension in these animals [4] , [5] , as has been observed in dietary-restricted C. elegans [6] , [7] . However, PHA-4/FOXA may not be a general transcriptional regulator of autophagy, because inhibition of PHA-4/FOXA has only a minor effect on the long lifespan of insulin/IGF-1 signalling mutants or animals with reduced mitochondrial respiration [6] . Thus, it is not clear whether induction of autophagy in these longevity pathways is mediated by a common transcriptional regulator. The basic helix-loop-helix (HLH) transcription factor EB (TFEB) was recently identified as a key transcriptional regulator of the autophagy process in mammals [8] . In mammalian cells, TFEB translocates to the nucleus in response to nutrient deprivation, at least in part, via a TOR-dependent mechanism [9] , [10] , [11] to ensure the transcriptional induction of many autophagy-related and lysosomal genes [8] . In this study, we asked whether C. elegans contains a functional orthologue of TFEB, and if so, whether the orthologue has a role in lifespan determination. To this end, we examined HLH-30 (W02C12.3, www.wormbase.org ), which is a member of a group of 42 HLH transcription factors in C. elegans and has the highest homology to TFEB in the DNA-binding domain and in an acidic activation domain [12] . We report that HLH-30 regulates the expression of multiple autophagy-related and lysosomal genes, and modulates the autophagy process in C. elegans. HLH-30 is required for the long lifespan observed in all C. elegans longevity mutants tested, is nuclear localized in these long-lived models, and the overexpression of HLH-30 extends the C. elegans lifespan. Taken together, these observations suggest that increased HLH-30 activity may be a universal mechanism for longevity. Finally, we find that TFEB levels are increased in the liver nuclear extracts of dietary-restricted mice, raising the possibility that HLH-30/TFEB modulates lifespan in a conserved manner. HLH-30 locates to the nucleus in animals with reduced TOR activity Our recent work showed that autophagy is transcriptionally activated in long-lived, germline-less C. elegans , such as temperature-sensitive glp-1/ Notch receptor mutants, possibly via a reduction in TOR activity [4] . Therefore, we used glp-1(e2141) mutants raised at the restrictive temperature to investigate whether HLH-30 has a role in autophagy regulation in C. elegans via TOR, as observed in mammalian cells [9] , [10] , [11] . Consistent with this possibility, we observed green fluorescent protein (GFP)-tagged HLH-30 to be enriched prominently in the nuclei of intestinal cells in adult glp-1(e2141) mutants ( Fig. 1 ). Similarly, we observed nuclear localization of HLH-30 in wild-type (WT; N2 Bristol) animals subjected to tor RNA interference (RNAi) ( Fig. 2 ). These observations suggest that HLH-30 localizes to the nucleus in C. elegans intestinal cells under conditions associated with induction of autophagy, including TOR inhibition, similar to TFEB in mammalian cells [9] , [10] , [11] . 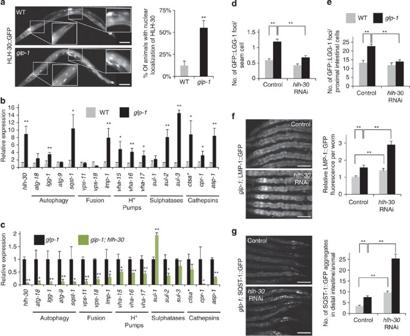Figure 1: HLH-30 regulates autophagy in germline-lessC. elegans. (a) Nuclear localization of HLH-30 was visualized by fluorescence microscopy in day 1 adult wild-type (WT) (upper panel) andglp-1(e2141)(lower panel) animals expressing HLH-30::GFP raised at the non-permissive temperature (25 °C). Inserts show enlarged intestinal cells. Graph shows percentage of animals with HLH-30 in the nuclei of intestinal cells (four biological replicates, ~50 animals each, mean±s.d., **P<0.01, Student’st-test). Magnification × 100; scale bar, 100 μm. (b) Expression ofhlh-30and putative autophagy-related and lysosomal target genes was measured by quantitative PCR (qPCR) in day 1 adult WT andglp-1(e2141)animals raised at 25 °C (mean±s.d. of three biological replicates, *P<0.05, **P<0.01, Student’st-test). (c) Expression ofhlh-30and putative autophagy-related and lysosomal target genes was measured by qPCR in day 1 adultglp-1(e2141)andglp-1(e2141);hlh-30(tm1978)animals raised at 25 °C (mean±s.d. of three biological replicates, *P<0.05, **P<0.01, Student’st-test).ctsa*is a cathepsin A orthologue (cosmid C08H9.1 (ref.30)). SeeSupplementary Fig. 1for qPCR analyses ofhlh-30(tm1978)(control forc) and WT andglp-1(e2141)animals fed bacteria expressinghlh-30dsRNA. (d,e) GFP::LGG-1 punctae were quantified in (d) hypodermal seam cells or (e) proximal intestinal cells of L3 larvae of WT andglp-1(e2141)animals. Animals were fed bacteria expressing control orhlh-30dsRNA for two generations at 20 °C. Eggs were then transferred to plates seeded with the appropriate dsRNA-expressing bacteria at 25 °C and analysed at the L3 larval stage (mean±s.e.m. of ~300 seam cells and ~25 intestines, **P<0.01, Student’st-test). (f,g)glp-1(e2141)animals expressing (f) LMP-1::GFP or (g) SQST-1::GFP were raised at the non-permissive temperature (25 °C) and fed bacteria expressing control orhlh-30dsRNA from hatching. Micrographs of the posterior intestine were taken on day 1 of adulthood, and LMP-1::GFP fluorescence (mean±s.d. of ~10 animals, **P<0.01, Student’st-test) and SQST-1::GFP foci (mean±s.d. of ~30 animals, **P<0.01, Student’st-test) were quantified. Experiments were performed at least three times with similar results. See Supplementary Fig. S2a,c for images of whole animals and Supplementary Fig. S2b,d for replicates. Magnification, × 200; scale bar, 100 μm. Figure 1: HLH-30 regulates autophagy in germline-less C. elegans . ( a ) Nuclear localization of HLH-30 was visualized by fluorescence microscopy in day 1 adult wild-type (WT) (upper panel) and glp-1(e2141) (lower panel) animals expressing HLH-30::GFP raised at the non-permissive temperature (25 °C). Inserts show enlarged intestinal cells. Graph shows percentage of animals with HLH-30 in the nuclei of intestinal cells (four biological replicates, ~50 animals each, mean±s.d., ** P <0.01, Student’s t -test). Magnification × 100; scale bar, 100 μm. ( b ) Expression of hlh-30 and putative autophagy-related and lysosomal target genes was measured by quantitative PCR (qPCR) in day 1 adult WT and glp-1(e2141) animals raised at 25 °C (mean±s.d. of three biological replicates, * P <0.05, ** P <0.01, Student’s t -test). ( c ) Expression of hlh-30 and putative autophagy-related and lysosomal target genes was measured by qPCR in day 1 adult glp-1(e2141) and glp-1(e2141) ; hlh-30(tm1978) animals raised at 25 °C (mean±s.d. of three biological replicates, * P <0.05, ** P <0.01, Student’s t -test). ctsa* is a cathepsin A orthologue (cosmid C08H9.1 (ref. 30 )). See Supplementary Fig. 1 for qPCR analyses of hlh-30(tm1978) (control for c ) and WT and glp-1(e2141) animals fed bacteria expressing hlh-30 dsRNA. ( d , e ) GFP::LGG-1 punctae were quantified in ( d ) hypodermal seam cells or ( e ) proximal intestinal cells of L3 larvae of WT and glp-1(e2141) animals. Animals were fed bacteria expressing control or hlh-30 dsRNA for two generations at 20 °C. Eggs were then transferred to plates seeded with the appropriate dsRNA-expressing bacteria at 25 °C and analysed at the L3 larval stage (mean±s.e.m. of ~300 seam cells and ~25 intestines, ** P <0.01, Student’s t- test). ( f , g ) glp-1(e2141) animals expressing ( f ) LMP-1::GFP or ( g ) SQST-1::GFP were raised at the non-permissive temperature (25 °C) and fed bacteria expressing control or hlh-30 dsRNA from hatching. Micrographs of the posterior intestine were taken on day 1 of adulthood, and LMP-1::GFP fluorescence (mean±s.d. of ~10 animals, ** P <0.01, Student’s t -test) and SQST-1::GFP foci (mean±s.d. of ~30 animals, ** P <0.01, Student’s t -test) were quantified. Experiments were performed at least three times with similar results. See Supplementary Fig. S2a,c for images of whole animals and Supplementary Fig. S2b,d for replicates. Magnification, × 200; scale bar, 100 μm. 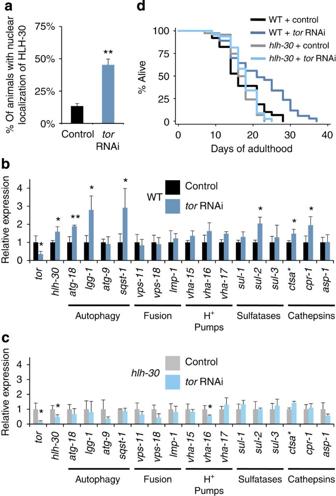Figure 2: HLH-30 is required for TOR inhibition to extendC. eleganslifespan. (a) Nuclear localization of HLH-30 was quantified in day 1 adult animals expressing HLH-30::GFP. Animals were fed bacteria expressing control ortordsRNA from hatching and raised at 20 °C (three biological replicates, ~50 animals each, mean±s.d., **P<0.01, Student’st-test). (b,c) Expression of putative autophagy-related and lysosomal target genes was measured by quantitative PCR in day 1 (b) WT (N2) and (c)hlh-30(tm1978)animals fed bacteria expressing control ortordsRNA from hatching (20 °C). Data are mean±s.d. of biological triplicates. *P<0.05, **P<0.01; Student’st-test.csta* is a cathepsin A orthologue (cosmid C08H9.1 (ref.30)).(d) Lifespan analysis of WT animals andhlh-30(tm1978)mutants fed bacteria expressing control ortordsRNA from day 1 of adulthood was carried out at 20 °C. SeeSupplementary Table S3for details of lifespan analyses and replicate experiments. Full size image Figure 2: HLH-30 is required for TOR inhibition to extend C. elegans lifespan. ( a ) Nuclear localization of HLH-30 was quantified in day 1 adult animals expressing HLH-30::GFP. Animals were fed bacteria expressing control or tor dsRNA from hatching and raised at 20 °C (three biological replicates, ~50 animals each, mean±s.d., ** P <0.01, Student’s t -test). ( b , c ) Expression of putative autophagy-related and lysosomal target genes was measured by quantitative PCR in day 1 ( b ) WT (N2) and ( c ) hlh-30(tm1978) animals fed bacteria expressing control or tor dsRNA from hatching (20 °C). Data are mean±s.d. of biological triplicates. * P <0.05, ** P <0.01; Student’s t -test. csta * is a cathepsin A orthologue (cosmid C08H9.1 (ref. 30 )). ( d ) Lifespan analysis of WT animals and hlh-30(tm1978) mutants fed bacteria expressing control or tor dsRNA from day 1 of adulthood was carried out at 20 °C. See Supplementary Table S3 for details of lifespan analyses and replicate experiments. Full size image HLH-30 regulates the expression of orthologous TFEB targets We next investigated the expression of hlh-30 and orthologues of TFEB target genes in glp-1(e2141) mutants and in WT animals with reduced TOR levels. We found that hlh-30 mRNA levels were markedly increased in both glp-1(e2141) and tor(RNAi) mutants when compared with WT animals ( Figs 1b and 2b ). Moreover, glp-1(e2141) mutants showed increased expression of several nematode orthologues of human TFEB target genes, including genes involved in autophagosome formation and autophagic flux, such as lgg-1 /LC3 and sqst-1/ SQSTM1/p62, and genes with lysosomal functions, such as lmp-1/ LAMP-1, subunits of vacuolar ATPases ( vha-15 , vha-16 and vha-17 ), sulphatases ( sul-2/ASRA and sul-3/ASRA ) and cathepsins ( ctsa/ cathepsin A, cpr-1/ cathepsin B and asp-1/ cathepsin D) ( Fig. 1b ). Several of these autophagy-related and lysosomal genes were similarly changed in adult WT animals subjected to tor RNAi ( Fig. 2b ). Changes in the expression of these genes may be transcriptionally regulated by hlh-30 , because glp-1(e2141); hlh-30(tm1978) double mutants or hlh-30(tm1978) single mutants fed bacteria expressing tor dsRNA, all showed a profound reduction in transcription of most of the putative target genes ( Figs 1c and 2c ). The glp-1(e2141) mutants fed bacteria expressing hlh-30 dsRNA only during adulthood showed decreased expression of most target genes ( Supplementary Fig. S1a ), whereas inhibition of hlh-30 by RNAi in WT animals had a modest or no effect on the expression of these genes ( Supplementary Fig. S1b ). We also found that hlh-30(tm1978) single mutants displayed decreased expression of some (for example, atg-18 ), but not all, of these genes ( Supplementary Fig. S1c ), consistent with a previously published microarray analysis [13] . Notably, most of the genes examined contain one or more E-box motifs in their promoters ( Supplementary Table S1 ); this sequence overlaps with that of the CLEAR (Coordinated Lysosomal Expression And Regulation) binding motif, which is present in the promoters of many lysosomal gene targets of TFEB [14] . Collectively, these data suggest that HLH-30 functionally mimics TFEB by inducing the transcription of autophagy-related and lysosomal genes. HLH-30 modulates autophagy and lysosomal function To directly determine whether HLH-30 regulates autophagy, we used transgenic WT and glp-1(e2141) animals expressing GFP reporters that allow distinct steps of the autophagy process to be examined. First, we used a strain expressing GFP-tagged LGG-1/LC3 (ref. 15 ), a protein that localizes to preautophagosomal and autophagosomal membranes, to investigate autophagosome formation. Compared with WT animals, glp-1(e2141) mutants contained more GFP::LGG-1-positive punctae, reflecting an increased number of autophagosomes [4] . However, significantly fewer GFP::LGG-1-positive punctae were detected in both hypodermal seam cells and intestinal cells of hlh-30 RNAi-treated glp-1(e2141) animals compared with that in control animals ( Fig. 1d, e ), suggesting that hlh-30 is required for autophagy induction in glp-1(e2141) mutants. To monitor the lysosomal compartment, we used a strain expressing GFP-tagged LMP-1/LAMP1 (ref. 16 ), a glycoprotein localized to the lysosomal membrane. Germline-less glp-1(e2141) animals displayed slightly elevated expression of LMP-1/LAMP1 ( Supplementary Fig. S2a ), indicative of enhanced lysosomal biogenesis. This is consistent with our previous observation that germline-less animals display increased autophagosome formation [4] . Notably, the expression of the LMP-1::GFP reporter was robustly increased in the absence of hlh-30 ( Fig. 1f and Supplementary Fig. S2b ), as would be expected following the impairment of autophagy turnover. Finally, to monitor autophagic flux we used a strain expressing GFP-tagged SQST-1/p62 (ref. 17 ), an adaptor protein that targets autophagic cargo for degradation. SQST-1 was expressed at low levels in adult animals, where it localized to distinct subcellular sites, referred to as foci. Interestingly, we found the number of SQST-1::GFP foci was modestly increased in certain tissues of glp-1(e2141) mutants, including in some intestinal cells ( Fig. 1g and Supplementary Fig. S2c ). This may reflect a higher steady-state level of cargo delivery to autophagosomes and increased autophagic flux in specific tissues of these animals. The number of SQST-1::GFP foci was significantly increased following hlh-30 RNAi treatment ( Fig. 1g and Supplementary Fig. S2d ), consistent with a block in autophagic turnover of SQST-1/p62. In glp-1 animals with reduced HLH-30 levels, the modest increase in the expression of both LMP-1/LAMP1 and SQST-1/p62 occurred, despite a marked reduction in their mRNA levels ( Supplementary Fig. S1b ), implying that HLH-30 is necessary for the turnover of these proteins. Taken together, these results indicate that inhibition of HLH-30 impairs the coordination of the autophagy process at several steps, and suggest that HLH-30 regulates autophagy in a manner similar to TFEB [8] . glp-1 and TOR mutants require HLH-30 for lifespan extension As we previously reported that several of the putative HLH-30-regulated genes are required for the long lifespan of glp-1 animals (for example, atg-18 and lgg-1 (ref. 4 )), we next determined whether HLH-30 has a role in C. elegans lifespan. We performed survival analyses on adult WT and glp-1 animals fed bacteria, expressing hlh-30 dsRNA. Although hlh-30 RNAi administered during adulthood did not affect the lifespan of WT animals, this treatment significantly shortened the long lifespan of glp-1(e2141) mutants ( Fig. 3 and Supplementary Table S2 ). Likewise, we found glp-1(e2141); hlh-30(tm1978) double mutants to have mean lifespans similar to hlh-30(tm1978) single mutants ( Supplementary Fig. S3a and Supplementary Table S2 ). In addition, RNAi-mediated inhibition of the lysosomal gene vha-16 , but not of lmp-1 , substantially reduced the long lifespan of glp-1(e2141) mutants ( Supplementary Fig. S3b-d and Supplementary Table S3 ), supporting the notion that a subset of HLH-30-regulated genes, with functions relevant to autophagy, may contribute to lifespan extension. 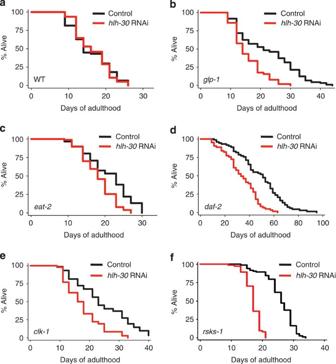Figure 3: HLH-30 is required for the long lifespan of multiple longevity mutants. Lifespan analyses of (a) WT (N2) and (b) germline-lessglp-1(e2141)animals raised at the non-permissive temperature (25 °C) and fed bacteria expressing control orhlh-30dsRNA from day 1 of adulthood were carried out at 20 °C. Lifespan analyses of (c) dietary-restrictedeat-2(ad1116)mutants, (d) insulin/IGF-1 receptordaf-2(e1370)mutants, (e) mitochondrial respirationclk-1(e2519)mutants and (f) mRNA translationrsks-1(sv31)mutants, fed bacteria expressing control orhlh-30dsRNA from day 1 of adulthood (c,d,f) or larval L4 stage (e), were carried out at 20 °C. SeeSupplementary Table S2for details of lifespan analyses including at least three independent experiments. Figure 3: HLH-30 is required for the long lifespan of multiple longevity mutants. Lifespan analyses of ( a ) WT (N2) and ( b ) germline-less glp-1(e2141) animals raised at the non-permissive temperature (25 °C) and fed bacteria expressing control or hlh-30 dsRNA from day 1 of adulthood were carried out at 20 °C. Lifespan analyses of ( c ) dietary-restricted eat-2(ad1116) mutants, ( d ) insulin/IGF-1 receptor daf-2(e1370) mutants, ( e ) mitochondrial respiration clk-1(e2519) mutants and ( f ) mRNA translation rsks-1(sv31) mutants, fed bacteria expressing control or hlh-30 dsRNA from day 1 of adulthood ( c , d , f ) or larval L4 stage ( e ), were carried out at 20 °C. See Supplementary Table S2 for details of lifespan analyses including at least three independent experiments. Full size image Similar to germline removal, reduced TOR activity extends lifespan at least partly via an autophagy-dependent mechanism [18] . To test whether hlh-30 has a role in TOR-mediated longevity in C. elegans , we fed bacteria expressing tor dsRNA to adult WT animals or mutants lacking hlh-30 bacteria. As expected, tor RNAi significantly extended the lifespan of WT animals; however, the same treatment failed to prolong the lifespan of hlh-30(tm1978) mutants ( Fig. 2d and Supplementary Table S4 ), suggesting that hlh-30 acts downstream of TOR. Consistent with this notion, we found that hlh-30 was required for the developmental arrest of C. elegans induced by treatment with tor RNAi for multiple generations ( Supplementary Fig. S4a, b ). Inhibition of hlh-30 also prevented dauer formation ( Supplementary Fig. S4c ), a developmental stage in which autophagy plays a critical role [15] , indicating that developmental arrest may be governed by hlh-30 , possibly via autophagy regulation. Taken together, these observations demonstrate that HLH-30 is a novel longevity-modulating transcription factor in C. elegans , which likely acts downstream of TOR. As HLH-30 regulates several autophagy-related genes with effects on longevity, it is possible that HLH-30 affects lifespan via regulation of autophagy in both germline-less animals and animals with reduced TOR function. HLH-30 is required for lifespan extension in other mutants In addition to germline removal and TOR inhibition, several other mechanistically distinct and conserved longevity pathways modulate aging in C. elegans : dietary restriction (DR; the feeding-deficient mutant eat-2 (ref. 19 )), inhibition of insulin/IGF-1 signalling (the receptor mutant daf-2 (ref. 20 )), impaired mitochondrial respiration (the ubiquinone synthesis mutant clk-1 (ref. 21 )) and reduced translation (the ribosomal S6 kinase mutant rsks-1 (refs 22 , 23 )). We therefore investigated whether hlh-30 has a role in lifespan determination in these longevity models. To do these experiments, we initiated hlh-30 RNAi during adulthood (for eat-2(ad1116) , daf-2(e1370) and rsks-1(sv31) mutants) or during the fourth larval stage (for clk-1(e2519) mutants). We found that hlh-30 RNAi significantly shortened the lifespan of these mutants ( Fig. 3c–f and Supplementary Table S2 ), suggesting a common role for HLH-30 in their longevity. To further investigate this possibility, we introduced the HLH-30::GFP transgene into eat-2 , daf-2 , clk-1 and rsks-1 mutants. Consistent with a regulatory role for hlh-30 , we observed that HLH-30 was nuclear localized in the intestine of eat-2(ad1116) , daf-2(e1370) , clk-1(e2519) and rsks-1(sv31) animals ( Fig. 4a ). Interestingly, although hlh-30 mRNA levels were significantly increased in these four long-lived mutants compared with WT animals ( Fig. 4b ), fewer of the TFEB target gene orthologues with functions in autophagy (for example, atg-9 ) were upregulated in eat-2(ad1116) , daf-2(e1370) , clk-1(e2519) and rsks-1(sv31) mutants ( Supplementary Fig. S6a ) than that in the glp-1(e2141) ( Fig. 1b ) and tor(RNAi) ( Fig. 2b ) mutants. These results suggest that HLH-30 may function differently in the distinct longevity mutants. As autophagy has been shown to have a role in the longevity of eat-2(ad1116) (refs 7 , 24 , 25 ), daf-2(e1370) (refs 7 , 15 , 26 ) and clk-1(e2519) ( Supplementary Table S5 ) mutants, and possibly also in rsks-1(sv31) mutants ( Supplementary Fig. S5 and Supplementary Table S6 ), these findings suggest that autophagy could be differentially regulated in the C. elegans longevity models. These results also indicate that HLH-30 may regulate additional genes with roles in longevity that are not necessarily related to autophagy. 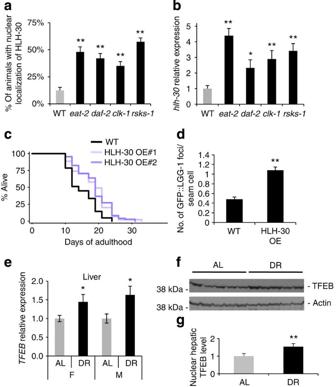Figure 4: HLH-30 and TFEB are similarly regulated in nematode and mouse longevity models. (a) Expression ofhlh-30was measured by quantitative PCR (qPCR) in day 1 adult WT (N2),eat-2(ad1116)(dietary restriction, DR),daf-2(e1370)(insulin/IGF-1 signaling),clk-1(e2519)(mitochondrial respiration) andrsks-1(sv31)(mRNA translation) animals (mean±s.d. of three biological replicates, *P<0.05, Student’st-test). (b) Nuclear localization of HLH-30 was quantified in day 1 adult WT,eat-2,daf-2,clk-1andrsks-1mutants (mean±s.d. of four biological replicates, ~50 animals each, **P<0.01, analysis of variance). (c) Lifespan analysis of WT and transgenic animals overexpressing HLH-30::GFP, and raised and maintained on OP50 was carried out at 20 °C. SeeSupplementary Table S7for details of lifespan analyses and replicate experiments. (d) GFP::LGG-1 punctae were quantified in hypodermal seam cells of WT animals or animals overexpressing HLH-30 (n>300, ±s.e.m., **P<0.01, Student’st-test). The increase in GFP::LGG-1 punctae observed in animals overexpressing HLH-30 could be reversed byatg-18RNAi treatment (data not shown). (e)TFEBexpression was measured by qPCR in the livers of 4.5-month-old female (F) and male (M) mice fed AL or subjected to DR for 5.5 weeks starting at 3 months of age (mean±s.e.m. of ~20 mice per group, *P<0.05, Student’st-test). (f) TFEB protein was detected by western blotting of nuclear fractions from the livers of five female and five male mice fed AL or subjected to DR. Actin was included as a loading control, seeSupplementary Fig. S8for additional controls. (g) TFEB protein levels inFig. 4fwere quantified by densitometry and normalized to actin (mean±s.d., *P<0.05, Student’st-test). Figure 4: HLH-30 and TFEB are similarly regulated in nematode and mouse longevity models. ( a ) Expression of hlh-30 was measured by quantitative PCR (qPCR) in day 1 adult WT (N2), eat-2(ad1116) (dietary restriction, DR), daf-2(e1370) (insulin/IGF-1 signaling), clk-1(e2519) (mitochondrial respiration) and rsks-1(sv31) (mRNA translation) animals (mean±s.d. of three biological replicates, * P <0.05, Student’s t -test). ( b ) Nuclear localization of HLH-30 was quantified in day 1 adult WT, eat-2 , daf-2 , clk-1 and rsks-1 mutants (mean±s.d. of four biological replicates, ~50 animals each, ** P <0.01, analysis of variance). ( c ) Lifespan analysis of WT and transgenic animals overexpressing HLH-30::GFP, and raised and maintained on OP50 was carried out at 20 °C. See Supplementary Table S7 for details of lifespan analyses and replicate experiments. ( d ) GFP::LGG-1 punctae were quantified in hypodermal seam cells of WT animals or animals overexpressing HLH-30 ( n >300, ±s.e.m., ** P <0.01, Student’s t -test). The increase in GFP::LGG-1 punctae observed in animals overexpressing HLH-30 could be reversed by atg-18 RNAi treatment (data not shown). ( e ) TFEB expression was measured by qPCR in the livers of 4.5-month-old female (F) and male (M) mice fed AL or subjected to DR for 5.5 weeks starting at 3 months of age (mean±s.e.m. of ~20 mice per group, * P <0.05, Student’s t -test). ( f ) TFEB protein was detected by western blotting of nuclear fractions from the livers of five female and five male mice fed AL or subjected to DR. Actin was included as a loading control, see Supplementary Fig. S8 for additional controls. ( g ) TFEB protein levels in Fig. 4f were quantified by densitometry and normalized to actin (mean±s.d., * P <0.05, Student’s t -test). Full size image Overexpression of HLH-30 extends C. elegans lifespan Our results indicated a requirement for hlh-30 in multiple C. elegans longevity models. To determine whether HLH-30 expression was sufficient to extend C. elegans lifespan, we generated strains stably overexpressing HLH-30::GFP from transgenic, integrated arrays and measured the lifespan of two independent lines. We observed that the mean lifespan of the transgenic animals was ~15–20% longer than that of WT animals ( Fig. 4c and Supplementary Table S7 ). These long-lived animals showed a partial induction of the genes regulated in glp-1(e2141) and tor(RNAi) mutants ( Supplementary Fig. S6b ), suggesting that the long life of HLH-30-overexpressing animals may be mediated through partially overlapping mechanisms. Notably, HLH-30-overexpressing animals had increased numbers of GFP-positive, LGG-1-positive punctae ( Fig. 4d ), and inhibition of the autophagy gene atg-18 reduced the lifespan of these animals ( Supplementary Table S8 ). Thus, HLH-30 may extend lifespan, at least in part, by inducing autophagy. Collectively, our data provide evidence that HLH-30 is a conserved transcription factor with a novel universal role in modulating C. elegans lifespan. Dietary restriction regulates TFEB in mice To determine whether TFEB, the mammalian orthologue of HLH-30, has a conserved role in lifespan determination, we asked whether TFEB is regulated under conditions that modulate longevity in mammals. For this, we examined mice placed on a dietary-restricted diet, an effective non-genetic intervention that extends lifespan in mammals [27] . In two key nutrient-responsive tissues, the liver and pancreas, we found TFEB mRNA levels to be significantly increased in male and female mice subjected to DR compared with control mice fed ad libitum (AL) ( Supplementary Fig. S8 ). Consistent with these observations, TFEB protein levels were also significantly higher in nuclear extracts of livers from dietary-restricted mice compared with control animals ( Fig. 4f ), as observed in all the long-lived C. elegans models we examined ( Figs 1a , 2b and 4b ). Taken together, these results raise the possibility that mammalian TFEB may have a broad and conserved role in lifespan extension. In this study, we show that the HLH transcription factor HLH-30 has a role in the determination of lifespan, and demonstrate that HLH-30 regulates autophagy in C. elegans , similar to the function of mammalian transcription factor TFEB [8] . Our studies reveal hlh-30 as a key transcription factor required for lifespan extension in all six longevity models analysed: germline removal, TOR inhibition, DR, reduced insulin/IGF-1 signalling, reduced mitochondrial respiration and reduced translation, suggesting a central role for HLH-30 in lifespan determination in C. elegans . Our results are consistent with HLH-30 being a functional orthologue of TFEB, because the expression of orthologues of many TFEB target genes with functions in multiple steps of the autophagy process were regulated by HLH-30 in both germline-less glp-1 mutants and animals with reduced TOR levels. Many of the conserved hlh-30 -regulated genes have predicted functions in autophagosome formation, cargo degradation, fusion and lysosomal degradation, including proton-translocating ATPases/pumps, and degradative enzymes, such as cathepsins and arylsulphatases. Thus, HLH-30 appears to display a broad role in the transcription of multiple genes with functions in several steps of the autophagy process. Consistent with this notion, the Ruvkun laboratory independently reported, while this study was under revision, a conserved role for HLH-30/TFEB in autophagy gene expression [28] . It remains to be investigated whether such HLH-30-regulated genes are direct or indirect targets of HLH-30. Our experiments with different reporter proteins indicated that induction of autophagosome formation and lysosomal degradation were impaired by the loss of hlh-30 , implying that HLH-30 regulates different stages of the autophagy process. We found that hlh-30 had a critical role in six mechanistically distinct C. elegans longevity models, many of which had previously been reported to rely, at least in part, on increased autophagy for their lifespan extension: germline ablation, TOR inhibition, DR, reduced insulin/IGF-1 signalling and reduced mitochondrial respiration. This may also be the case for animals with reduced levels of the S6 kinase RSKS-1, as we found that the long lifespan of these animals was dependent on at least one autophagy gene, atg-18 , and we observed an increase in autophagic events in adult animals ( Supplementary Fig. S5 ). The observation that hlh-30 is upregulated and is required for the long lifespan in these C. elegans longevity paradigms is notable, because no downstream transcription factor common to these models has so far been described. In addition, the Ruvkun and Ballabio laboratories recently reported that hlh-30 is required for lifespan extension induced by a loss-of-function mutation of the transcription factor mxl-3 (Max-like 3) [28] and for starvation-induced longevity [29] in C. elegans . Although it remains to be investigated how these mechanistically different longevity models activate HLH-30, TOR regulation is a candidate mechanism [9] , [10] , [11] , [28] . The identification of HLH-30 as a key transcription factor that regulates multiple genes with functions throughout the autophagy process supports the concept that increased autophagic flux is likely critical to ensure long lifespan. Indeed, we found that knockdown of vha-16 , a lysosomal ATPase, significantly shortened the long lifespan of germline-less glp-1 animals, as previously observed for genes important for early steps in the autophagy process [4] . Another lysosomal gene, C08H9.1/cathepsin A was previously reported to be required for the long lifespan of daf-2 /insulin/IGF-1 mutants [30] , supporting the notion that lysosomal function has an important role in distinct longevity mechanisms. Nonetheless, knockdown of the lysosomal glycoprotein lmp-1 did not shorten glp-1 -mediated lifespan extension, implying that not all lysosomal hlh-30 -regulated genes contribute to lifespan. Although our data are consistent with HLH-30 mediating lifespan extension in multiple longevity pathways, at least in part, by inducing autophagy, it is possible that other HLH-30-regulated mechanisms, such as lipid metabolism [28] , [29] , are also concomitantly engaged. As C. elegans longevity pathways engage distinct sets of transcription factors [1] , it will also be interesting to investigate how the activities of HLH-30 and other lifespan-modulating transcription factors, for example, PHA-4/FOXA [4] , [6] , are coordinated in specific longevity models. We found that at least two aspects of C. elegans HLH-30 function were conserved in a mammalian model of longevity, namely, DR [27] . Expression of TFEB was increased in the pancreas and liver of dietary-restricted mice, tissues known to respond to starvation by autophagy induction [31] , and nuclear TFEB protein levels were enhanced in the livers from dietary-restricted mice. It will be interesting to investigate the transcriptional activity of TFEB in response to DR in mammals. Taken together, these results support the intriguing possibility that TFEB might have a conserved role in lifespan modulation in higher organisms. In conclusion, our study demonstrates novel, essential and, possibly, conserved roles for the transcription factor HLH-30/TFEB in modulation of longevity by mechanisms that rely, at least partly, on the autophagy process. HLH-30 is the first transcription factor reported to function in all known autophagy-dependent C. elegans longevity paradigms, strengthening the emerging concept that increased autophagy can contribute to long lifespan. Accumulating evidence suggests that failure of the autophagy–lysosomal pathway contributes to the pathogenesis of a variety of age-related disorders [32] , [33] . Thus, HLH-30 and TFEB may represent attractive targets for the development of therapeutic agents for such diseases. Animals C. elegans strains (a list is available in Supplementary Table S9 ) were maintained on OP50 Escherichia coli at 20 °C and were handled using standard methods [34] . All mice procedures were carried out ethically according to the guidelines of the Institutional Animal Care and Use Committee Conduct and have been approved by the Salk Institute Institutional Animal Care and Use Committee Conduct Department. Construction of HLH-30 transgenic strains An expression plasmid for hlh-30p :: hlh-30::gfp was created by Gateway cloning technology lambda (Gateway System, Life Technologies) using pDONR P4-P1R- hlh-30p (2 kb promoter, Open Biosystems, Vidal promoterome library), pDONR201- hlh-30 open reading frame (Vidal ORFeome library, isoform W02C12.3a) and pKA674/pDEST-MB14-GFP destination vector (a generous gift from Kaveh Ashrafi, UCSF). Upon sequencing of the hlh-30 open reading frame, the codons for amino acids 123 and 255 were found to diverge from the corresponding RefSeq file (NP_500462.1) and were restored to the WT sequence using a QuikChange Site-Directed Mutagenesis kit (Agilent Technologies, Santa Clara, CA). Transgenic animals expressing an extra-chromosomal array of hlh-30p::hlh-30::gfp were created by gonadal microinjection of the plasmid pKA674( hlh-30p::hlh-30::gfp ) (10 ng μl −1 ) into young gravid adult WT animals using pRF4/ rol-6(su1006) (100 ng μl −1 ) as a selection marker. Integration was subsequently performed by γ-irradiation, followed by outcrossing four times to N2 WT animals. The nuclear localization of HLH-30::GFP was visualized with a Leica fluorescence dissecting scope equipped with a Leica DFC310 FX camera in animals within 5 min of mounting on a 2% agarose pad, because HLH-30::GFP translocates to the nucleus during starvation and under stress caused by mounting (data not shown). Autophagy measurements Animals expressing GFP::LGG-1 were synchronized and raised at the appropriate temperature on media plates seeded with bacteria expressing control or hlh-30 dsRNA. For the HLH-30-overexpressing animals, heterozygous F1 progeny from cross between strains MAH236 and MAH240 (see Supplementary Information ) was analysed. The number of GFP::LGG-1 punctae were counted in seam and intestinal cells at L3–L4 larval stage as described [4] . Worms were analysed at × 1,000 magnification on a Zeiss Imager Z1 after mounting on a 2% agarose pad in M9 medium containing 0.1% NaN 3 . SQST-1::GFP foci and LMP-1::GFP signal were imaged in animals on media plates with a Leica DFC310 FX camera. SQST-1::GFP foci were counted visually in the posterior intestine (from vulva to the tail), and LMP-1::GFP fluorescence was quantified using ImageJ 1.45 software (National Institute of Health, Bethesda, MD). Statistical analysis was done using GraphPad Prism 5.0 (GraphPad, La Jolla, CA). Quantification of GFP::LGG-1 punctae by confocal microscopy Day 1 adult WT or rsks-1(sv31) animals expressing GFP::LGG-1 fed OP50 E. coli bacteria and grown at 20 °C were mounted on a 2% agarose pad containing 0.1% 1.5 M NaN 3 . Worms were imaged using a LSM Zeiss 710 scanning confocal microscope. Z -stacks were taken at 0.6-μm slices. GFP excitation/emission was limited to 493/512 nm to eliminate background autofluorescence from the worms. Four experiments with 10–15 L3 worms or day 1 adults were imaged for each experiment. The number of GFP::LGG-1-positive punctae were counted in the seam cells, intestinal cells and muscle in one 0.6 μm slice. The Z -position of the seam cells and intestinal cells was chosen at a position where the nucleus could be clearly seen. Statistical analysis (analysis of variance) was performed with GraphPad Prism 5.0 software (GraphPad, La Jolla, CA). Lifespan analysis Synchronized animals, raised at 20°C and fed OP50 E. coli until adulthood, were transferred onto plates seeded with RNAi clones from the Ahringer library [35] and viability was measured every 2–3 days, as described [36] . ~100 animals were tested in each experiment. The plasmid expressing dsRNA against let-363 (tor) was previously described [37] . Statistical analysis (log-rank) was performed with STATA (StataCorp, College Station, TX). Quantitative PCR in C. elegans Synchronized animals were raised at 20 °C, unless otherwise noted, and fed OP50 E. coli bacteria until they reached adulthood. For each strain, animals were collected with M9 solution at day 1 of adulthood for analysis. For RNAi experiments, wild-type (N2, WT) and glp-1(e2141) animals were raised at 25 °C on OP50 E. coli bacteria and were transferred onto plates freshly seeded with control bacteria or bacteria expressing dsRNA against the gene of interest. Animals were incubated at 20 °C for 48 h, then collected and washed twice with M9 solution. Nematodes (~1,000) were flash frozen in liquid N 2 and RNA was extracted with Trizol (Invitrogen/Life Technologies, Carlsbad, CA) as described [38] . Concentration and purity of RNA samples were determined with a NanoDrop spectrophotometer and samples were stored at −80 °C. Reverse transcription was performed on 1 μg RNA per sample using iScript Supermix (Bio-Rad, Hercules, CA). Samples were diluted 1/100 and complementary DNA standards (1/25–1/400) were prepared as serial dilutions from a mixture of the relevant cDNAs. Diluted samples and custom-designed primers (IDT, San Diego, CA) were mixed with SYBR Green (Roche, Indianapolis, IN) and samples were analysed using a Roche LightCycler 480 (Roche). Relative mRNA levels of target genes were normalized against the geometric mean [39] of the housekeeping genes act-1 , cyn-1, cdc-42 and pmp-3. Primer sequences can be found in Supplementary Table S10 . Nematode orthologues of the TFEB target genes analysed in this study were selected based on their significance in previous studies [8] , [14] . Each biological sample was analysed in duplicate or triplicate for each gene assayed. The mRNA levels of nematode genes are presented as mean±s.d. and statistical analysis of biological triplicates was performed by two-tailed Student’s t -test or analysis of variance using GraphPad Prism 5.0 software (GraphPad, La Jolla, CA). Quantitative PCR in mice Three-month-old C57BL/6 J male and female mice were subjected to short-term DR according to previously described methods [40] , [41] . The animal room was maintained at 22 °C on a 12:12 h light:dark cycle. Mice were housed individually and were allowed water AL throughout the experiment. All mice were initially fed with AIN-93 M AL pellets (Bio-Serv, Frenchtown, NJ). After 1 week of habituation, daily food intake was measured for each mouse over a period of 10 days. Hypophagic or hyperphagic mice were excluded from the study, and the remaining mice were randomly assigned to an AL group that had free access to standard AIN-93 M AL pellets, or to a DR group that received AIN-93 40% pellets (Bio-Serv) in an amount corresponding to 60% of their regular daily food intake. DR animals were fed once daily at 1800, h. Body weights were monitored to confirm the efficiency of DR and, as expected, body weight loss in both genders stabilized after 2.5 weeks of DR. The DR or AL feeding regimens were continued for further 3 weeks. On the day of killing, food was removed from cages of mice fed AL at 1100, h to minimize intragroup variation related to food intake, and mice from both groups were killed between 1500 and 1600, h by isoflurane anaesthesia followed by decapitation. Organs were collected immediately after death, snap-frozen in liquid nitrogen and were stored at −80 °C until analysis. Total RNA was extracted from frozen mouse tissues using the Qiazol/chloroform method and RNeasy columns (Qiagen, Valencia, CA). In brief, frozen tissues were grounded and homogenized in Qiazol using RNA/DNAse-free disposable pestles (VWR, San Francisco, CA). After chloroform extraction, the RNA-containing phase was transferred to RNeasy columns and RNA purification was achieved following the manufacturer’s instructions. RNA purity and concentration were determined on a NanoDrop spectrophotometer and samples were stored at −80 °C. Reverse transcription was performed with 1 μg of RNA per sample using the Qiagen Quantitect Reverse Transcription kit (Qiagen), according to the manufacturer’s recommendations. For quantitative PCR (qPCR), cDNAs were diluted 1/20 and mixed with the relevant primers (see Supplementary Table S10 ) and SYBR Green. qPCR was performed using the standard curve method on cDNAs from 10 females and 11 males in the AL group and 9 females and 10 males in the DR group. All biological samples were tested in triplicate (technical repeats) for each gene. Expression of TFEB was normalized to the geometric mean of RPL23 and ARBP housekeeping genes. We validated the use of the housekeeping genes in our experimental conditions using Normfinder and Genorm algorithms [42] . Normal distribution of data was verified by the Kolmogorov–Smirnov test, and groups were compared by two-tailed Student’s t -test using GraphPad Prism 5.0. (GraphPad, La Jolla, CA) Western blots of nuclear extracts from mice Nuclear extraction was performed on 100 mg of snap-frozen liver from DR and AL-fed mice using the Active Motif nuclear extraction kit (Active Motif, Carlsbad, CA) following manufacturer instructions. Nuclear protein concentration was measured using a BCA kit (Thermo Scientific Pierce, Rockford, IL) and 50 μg protein from each sample were resolved on a 4–12% Bis-Tris precast gel (Invitrogen, Carlsbad, CA), and subsequently transferred to a polyvinylidene difluoride membrane. Blocking was performed for 1 h in 5% BSA. Antibodies used were mouse anti-TFEB antibody (My Biosource, MBS120432, San Diego, CA) diluted to 1/200, mouse anti-tubulin (T5168, Sigma, St Louis, MO) diluted to 1/5,000, and mouse anti-actin (Millipore, Billerica, MA), catalogue Number MAB1501R) diluted to 1/1,000 in PBS–BSA 5%–Tween 0.1%. After overnight 4 °C incubation with primary antibody, washes were done in PBS–Tween 0.1% and species-specific secondary antibody conjugated to horseradish peroxidase (Bio-Rad) were applied for 1 h and revealed with ECL reagent (Thermo Scientific Pierce, Rockford, IL). Quantification of nuclear TFEB and nuclear actin [43] was performed using ImageJ, and two-tailed Student’s t -test were done using GraphPad Prism 5.0. How to cite this article: Lapierre, L. R. et al . The TFEB orthologue HLH-30 regulates autophagy and modulates longevity in Caenorhabditis elegans . Nat. Commun. 4:2267 doi: 10.1038/ncomms3267 (2013).